Is wave–particle objectivity compatible with determinism and locality? Wave–particle duality, superposition and entanglement are among the most counterintuitive features of quantum theory. Their clash with our classical expectations motivated hidden-variable (HV) theories. With the emergence of quantum technologies, we can test experimentally the predictions of quantum theory versus HV theories and put strong restrictions on their key assumptions. Here, we study an entanglement-assisted version of the quantum delayed-choice experiment and show that the extension of HV to the controlling devices only exacerbates the contradiction. We compare HV theories that satisfy the conditions of objectivity (a property of photons being either particles or waves, but not both), determinism and local independence of hidden variables with quantum mechanics. Any two of the above conditions are compatible with it. The conflict becomes manifest when all three conditions are imposed and persists for any non-zero value of entanglement. We propose an experiment to test our conclusions. Quantum mechanics is proverbially counterintuitive [1] , [2] . For many years, thought experiments were used to dissect its puzzling properties, while hidden-variable (HV) models strived to explain or even to remove them [1] , [2] , [3] , [4] . The development of quantum technologies [5] , [6] enabled us not only to perform several former gedanken experiments [1] , [2] , but also to devise new ones [7] , [8] , [9] , [10] , [11] . One can gain new insights into quantum foundations by introducing quantum controlling devices [10] , [11] , [12] into well-known experiments. This has led, for example, to a reinterpretation [11] , [12] , [13] , [14] of Bohr’s complementarity principle [15] . Wave–particle duality is best illustrated by the classic Wheeler delayed-choice experiment (WDC) [16] , [17] , [18] , Fig. 1a,b . A photon enters a Mach–Zehnder interferometer (MZI) and its trajectory is coherently split by the beamsplitter BS 1 into an upper and a lower path. The upper path contains a variable phase shift ϕ . A random number generator controls the insertion ( b =1) or removal ( b =0) of a second beamsplitter BS 2 . If BS 2 is present, the interferometer is closed and we observe an interference pattern depending on the phase shift ϕ . If BS 2 is absent, the MZI is open and the detectors measure a constant probability distribution independent of ϕ . Thus, depending on the experimental setup, the photon behaves in two completely different ways. In the case of the closed MZI, the interference pattern suggests that the photon travelled along both paths simultaneously and interfered with itself at the second beamsplitter BS 2 , hence showing a wave-like behaviour. However, if the interferometer is open, since always only one of the two detectors fires, one is led to the conclusion that the photon travelled only one path, hence displaying a particle-like behaviour. 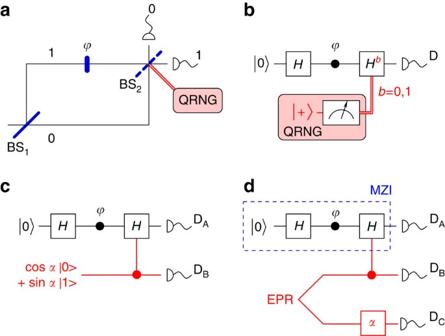Figure 1: The evolution of the delayed-choice experiment. (a) In Wheeler’s classic experiment, the second beamsplitter is inserted or removed after the photon is inside the interferometer; this prevents the photon from changing its mind16about being a particle or a wave. The detectors observe either an interference pattern depending on the phaseφ(wave behaviour), or an equal distribution of hits (particle behaviour). A quantum random number generator (QRNG) determines whether BS2is inserted or not. Quantum networks: (b) in the classic delayed-choice experiment the QRNG is an auxiliary quantum system initially prepared in the equal superposition stateand then measured. The Hadamard gateHis the quantum network equivalent of the beamsplitter; (c) delayed choice with a quantum control11; (d) entanglement-assisted quantum delayed-choice experiment19. The ancilla C is measured along the direction −α, equivalent to the application of a rotationbefore a measurement in the computational basis. Figure 1: The evolution of the delayed-choice experiment. ( a ) In Wheeler’s classic experiment, the second beamsplitter is inserted or removed after the photon is inside the interferometer; this prevents the photon from changing its mind [16] about being a particle or a wave. The detectors observe either an interference pattern depending on the phase φ (wave behaviour), or an equal distribution of hits (particle behaviour). A quantum random number generator (QRNG) determines whether BS 2 is inserted or not. Quantum networks: ( b ) in the classic delayed-choice experiment the QRNG is an auxiliary quantum system initially prepared in the equal superposition state and then measured. The Hadamard gate H is the quantum network equivalent of the beamsplitter; ( c ) delayed choice with a quantum control [11] ; ( d ) entanglement-assisted quantum delayed-choice experiment [19] . The ancilla C is measured along the direction − α , equivalent to the application of a rotation before a measurement in the computational basis. Full size image The complementarity of the interferometer setups required to observe particle or wave behaviour obscures the simultaneous presence of both properties, allowing the (objective) view that, at any moment of time, a photon can be either a particle or a wave. The WDC experiment uncovers the difficulty inherent in this view by randomly choosing whether or not to insert the second beamsplitter (BS 2 ) after the photon enters the interferometer ( Fig. 1a ). This delayed choice prevents a possible causal link between the experimental setup and the photon’s behaviour: the photon should not know beforehand if it has to behave like a particle or like a wave. The delayed-choice experiment with a quantum control ( Fig. 1c ) highlights the complexity of space–time ordering of events, once parts of the experimental setup become quantum systems [11] . The quantum-controlled delayed-choice experiment has been recently implemented in several different systems [19] , [20] , [21] , [22] , [23] . To ensure the quantum behaviour of the controlling device, one can either test the Bell inequality [23] or use an entangled ancilla [19] . The theoretical analysis of the quantum WDC involved so far a single binary HV λ describing the classical concepts of wave/particle. Here, we introduce a full HV description for both the photon A and the ancilla. We analyse the relationships between the concepts of determinism, wave–particle objectivity and local independence of HV in the entanglement-controlled delayed-choice experiment. We show that, when combined, these assumptions lead to predictions that are different from those of quantum mechanics, even if any two of them are compatible with it. We propose and discuss an experiment to test our conclusions. Notation We use the conventions as in refs 3 , 12 ; q ( a , b ,…) are the quantum-mechanical probability distributions and p ( a , b , . . . , Λ) the predictions of HV theories with a HV Λ. We consider either a single HV Λ, which fully determines behaviour of the system, or refine it as Λ 1 , Λ 2 pertaining to different parts of the system. For simplicity, we assume Λ is discrete; the analysis can be easily generalized to the continuous case. Quantum system The system we analyse consists of three qubits: a photon A and an entangled pair BC ( Fig. 1d ). We denote the measurement outcomes for the photon A as a =0, 1 and for the two ancilla qubits as b and c ; the corresponding detectors are D A , D B and D C . The system is prepared in the initial state ; for , BC is a maximally entangled EPR pair. Photon A enters a MZI in which the second beamsplitter is quantum-controlled by qubit B. The third qubit C undergoes a σ y rotation followed by a measurement in the computational basis. The state before the measurements is The counting statistics that result from the particle-like state and the wave-like state are discussed below (equations (3 and 4) and Methods). Constraints on HV theories Our strategy is to show that q ( a , b , c ) cannot result from a probability distribution p ( a , b , c , Λ) of a HV theory satisfying the requirements of wave–particle objectivity, local independence and determinism. Any viable HV theory should satisfy the adequacy condition: namely, it should reproduce the quantum statistics by summing over all HVs Λ: We encapsulate the additional classical expectations into three assumptions (see Box 1 for the formal definitions of the concepts we consider in this section). For a given photon, we require the property of being a particle or a wave to be objective (intrinsic), that is, to be unchanged during its lifetime. This condition selects from the set of adequate HV theories those models that have meaningful notions of particle and wave [11] . For each photon, the HV Λ should determine unambiguously if the photon is a particle or a wave, thus allowing the partition of the set of HVs into two disjoint subsets, = p ∪ w , where the subscript indicates the property, particle or wave. The particle (wave) properties are abstractions of the particle (wave) counting statistics in open (closed) MZI, respectively. The behaviour of a particle (wave) in a closed (open) MZI is not constrained; this allows for significant freedom in constructing HV theories. Experimentally, the wave or particle behaviour depends only on the photon and the settings of the MZI: for all values of a , b , c and Λ. By replacing the single-qubit ancilla with an entangled pair, one can take advantage of both the quantum control and the space-like separation between events. The rationale behind the third qubit C is that it allows us to choose the rotation angle α after both qubits A (the photon) and B (the quantum control) are detected. This is not possible in the standard quantum WDC [11] , Fig. 1c , where the quantum control B has to be prepared (by setting the angle α ) before it interacts with A. As discussed in Methods, there is a unique assignment of probabilities that satisfies all the requirements of adequacy, wave–particle objectivity and determinism. Adopting this assignment, we reach the same level of incongruity as in ref. 11 , since the probability p ( λ ) of photon A being a particle or a wave is determined by the entanglement between B and C, This incongruity becomes an impossibility when the photon A and the entangled pair BC are prepared independently. In this case, their HVs are generated independently; that is, a single HV Λ not only has the structure Λ=(Λ 1 ,Λ 2 ), where the subscripts 1 and 2 refer to the photon A and the pair BC, respectively, but the prior probability distribution of HV has a product form. To realize this condition experimentally, we rely on the absence of the superluminal communication and a space-like separation of the two events. Unlike the typical Bell-inequality scenarios, we have a single measurement setup which involves two independent HV distributions. Moreover, by performing the rotation R y ( α ) and the detection D C sufficiently fast, such that the information about A and Λ 1 cannot reach the detector D C , the detection outcome is determined only by Λ 2 . Since being a wave (particle) is assumed to be an objective property of A, λ = λ (Λ 1 ) is a binary function of the HV Λ 1 only. Box 1: Wave–particle objectivity . We define particles and waves according to the experimental behaviour in an open, respectively closed, MZI [11] . A particle in an open interferometer ( b =0) is insensitive to the phase shift in one of the arms and therefore has the statistics In contrast, a wave in a closed MZI ( b =1) shows interference The sets p and w must be disjoint; otherwise, there are values of Λ that introduce wave–particle duality. Writing p ∪ w = , the wave/particle property is expressed by a mapping λ : ↦ { p , w} and the sets p = λ −1 ( p ), w = λ −1 (w) are the pre-images of p , w under the function λ . Determinism . The HV Λ determines the individual outcomes of the detection [3] . Specifically, for the setup of ( Fig. 1d ) where the indicator function χ =1, if Λ belongs to some predetermined set, and χ =0 otherwise. Local independence . The HV Λ are split into Λ 1 and Λ 2 , and the prior probability distribution has a product structure for some probability distributions f and F , where the subscripts 1 and 2, respectively, refer to the photon A and the pair BC. Such bilocal variables have been previously considered in ref. 29 . Contradiction We show in Methods that for η ≠0, 1 (these two cases correspond to an always closed or opened MZI), the requirements of adequacy, wave–particle objectivity, determinism and local independence are satisfied only if This proves our main theoretical result: determinism, local independence and wave–particle objectivity are not compatible with quantum mechanics for any α ≠± π /4, ±3 π /4. We will later discuss how exactly a HV theory that satisfies the three classical assumptions is inadequate. Proposed experiment In Fig. 2 , we show the proposed experimental setup for the entanglement-controlled delayed-choice experiment. Two pump pulses (blue) are incident on two nonlinear crystals and generate via spontaneous parametric down-conversion two pairs of entangled photons (red). One of the photons is the trigger and the other three are the photons A, B, C, with BC being the entangled pair. 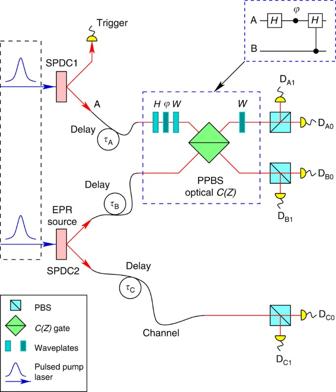Figure 2: Proposed experimental setup. Two space-like separated pump pulses (blue) generate, via spontaneous parametric down-conversion, two pairs of entangled photons (red). The first photon is the trigger and the other three the photons A, B, C. Inset: the quantum-controlled MZI. The optical delays in the three photon arms,τA,τB,τCcan be adjusted to ensure the desired time ordering of the detection events. Figure 2: Proposed experimental setup. Two space-like separated pump pulses (blue) generate, via spontaneous parametric down-conversion, two pairs of entangled photons (red). The first photon is the trigger and the other three the photons A, B, C. Inset: the quantum-controlled MZI. The optical delays in the three photon arms, τ A , τ B , τ C can be adjusted to ensure the desired time ordering of the detection events. Full size image Photons A and B are held in the lab (with appropriate delay lines) and together they implement the controlled MZI. The central element is the quantum switch, which is the controlled-Hadamard gate C ( H )=( W ⊗ I ) C ( Z )( W ⊗ I ), where . The photonic controlled- Z gate C ( Z ) is implemented with a partially polarizing beamsplitter and is done probabilistically via post-selection [24] , [25] . Optical wave plates perform single-qubit rotations (gates H , ϕ and W ) on photon A. Photon C is sent through a channel at a distant location, then measured in a rotated basis. Two independent lasers generate the two photon pairs ( Fig. 2 (refs 26 , 27 )); in this case, we can use equation (6) to describe independent probability distributions for Λ 1 and Λ 2 . In this section, we consider how exactly a HV theory, which satisfies the three classical assumptions, fails the adequacy test. The interference pattern measured by the detector D A0 is I A ( ϕ )=Tr( ρ A |0〉〈0|), with ρ A =Tr BC | ψ 〉〈 ψ |, the reduced density matrix of photon A. The data can be postselected according to the outcome c resulting in I A| c . The visibility of the interference pattern (Methods) is V =( I max − I min )/( I max + I min ), where the min/max values are calculated with respect to ϕ . The postselected visibility for c =0 is ( Fig. 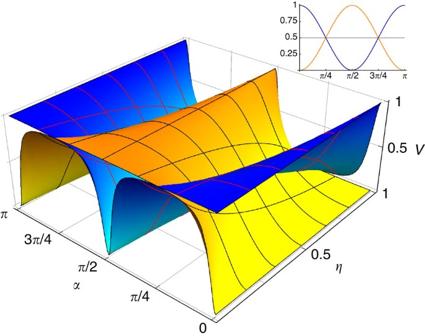Figure 3: Visibility. The visibilitiesVA|c=0(yellow) andVA|c=1(blue), are calculated in Methods. In HV theories, the visibility does not distinguish between thec=0, 1 cases. The inset illustrates this for, with the straight line representing the HV visibility prediction. 3 ) Figure 3: Visibility. The visibilities V A| c =0 (yellow) and V A| c =1 (blue), are calculated in Methods. In HV theories, the visibility does not distinguish between the c =0, 1 cases. The inset illustrates this for , with the straight line representing the HV visibility prediction. Full size image The full (non-postselected) visibility is V A =1− η and gives information about the initial entanglement of the BC pair. On the other hand, if one assumes that the HV are distributed according to equation (6) and satisfy the wave–particle objectivity and determinism, the visibility is independent of c , in contrast with the quantum-mechanical prediction ( Fig. 3 ). Details of this calculation are in Methods. This incompatibility between the basic tenets of HV theories and quantum mechanics has two remarkable features. First, the contradiction is revealed for any, arbitrarily small, amount of entanglement. This test is in sharp distinction with Bell-type experiments insofar as our result is free from inequalities. Wave–particle objectivity, revealed only statistically, is more intuitive and technically milder than the assumption of sharp values of quantum incompatible observables. Second, in our setup, any two of the classical ideas together are compatible with the quantum-mechanical predictions. This fact, and the way we arrived at the contradiction, invite questions concerning the internal consistency of classical concepts [28] . Quantum-mechanical analysis The initial state of photons A, B and C is The ancilla qubits B and C are maximally entangled for . The final state before measurement is given by equation (1). From it, we calculate the quantum statistics q ( a , b , c ), where each of a , b , and c take the values {0, 1}. The probability distribution for c =0 is where the four entries correspond to the values ( a , b )=(00, 01, 10, 11). For c =1, we obtain This in turn yields For the probability distributions for b and c are equal. If , B and C are no longer maximally entangled and the symmetry between them is broken: a rotation α on C no longer corresponds to a rotation α on B. The conditional probabilities are and from Bayes’ rule q ( b | c )= q ( c | b ) q ( b )/ q ( c ). Solution to the three constraints We now show that it is possible to construct a HV model that is adequate, objective and deterministic. The unknown parameters at our disposal are 16 probabilities p ( a , b , c , λ ). These probabilities are derived from the underlying distribution p (Λ) summed over appropriate domains. At this stage, we do not enquire about the connection with the HV Λ. The probabilities p ( a , b , c , λ ) satisfy seven adequacy constraints, equations (13) and (14), plus the normalization constraint. The adequacy conditions can be written as In addition, equation (7) and the standard rules for the conditional probabilities, such as imply the existence of four additional constrains, The resulting linear system has a four-parameter family of solutions. However, a straightforward calculation shows that for all these solutions p 4 ( a , b , c , λ ), the resulting statistics in an open/closed MZI is independent of λ , that is, the statistics of D A is determined solely by the state of the interferometer. We can avoid the reintroduction of wave–particle duality using a special solution which imposes the b – λ correlation (compare ref. 11 ). As a result, and since the probabilities are positive, the eight above probabilities are zero individually. The system appears overconstrained, but it still has a unique solution In particular, Deriving the contradiction In addition to the partition of according to the values of λ =p, w, we will use the decomposition of the set of HV according to the outcomes of D C . The two branches c =0, 1 correspond to the partition where for Λ ∈ c , the outcome of D C is c . The assumption of local independence implies a Cartesian product structure of the set of HV, where the subsets depend on the experimental setup. When the superscripts 1 and 2 on are redundant, we may omit them. Now, we show that under the assumptions of adequacy and the three classical assumptions of the wave–particle objectivity, determinism and local independence, it is impossible to derive the solution p ( a , b , c , λ ) with any arrangement of the probabilities p (Λ). The probability of the outcome c satisfies To simplify the calculations, we enumerate the variables Λ 1,2 by the indices i , j , respectively. The domain corresponds, according to the hypothesis, to the index set J c of Λ 2 , and the domains and to the index sets I p and I w of Λ 1 , respectively. In particular, for some . The prior distribution of HV and the domains of summation can depend on the parameters η , ϕ and α . The putative behaviour of a wave ( λ =w) in an open ( b =0) interferometer and of a particle ( λ =p) in a closed ( b =1) one is characterized by two unknown distributions x ij , i ∈ I w and y ij , i ∈ I p , respectively allowing for a possible dependence on a value of Λ 2 . The remaining two sets of variables are the probability distributions for b conditioned on the values of HVs Λ: The requirement of adequacy means that the proposed HV theory reproduces the quantum statistics given above. For compactness, we refer to the probability of having the HV values , , as p ij , using the same convention as for x ij , y ij , z ij and υ ij . For c =0, we have with analogous expressions for c =1. Adding and subtracting equations (39) and (41) we obtain, respectively Adding equations (40) and (42) yields which on substitution back into equation (40) results in Four additional equations (giving a total of seven independent equations) are obtained for j ∈ J 1 with cos 2 α ↔sin 2 α . From equation (26), it follows that υ ij =0, i ∈ I w and z ij =1, i ∈ I p . Hence, for c =0, only two equations are not automatically satisfied, The corresponding equations for c =1 are which are in agreement with q ( c ), equation (18). Now we use the product structure of the probability distribution, equation (6), Using equations (28) and (30), we find that Adding the pairs of equations in (47) and (48) and summing over the index i , we express the adequacy condition , but on the other hand, for η ≠0, 1 summing over i in each of these four equations separately and using equation (50) we get These equations can be satisfied for any η only if resulting in the contradiction (for arbitrary α ) cos 2 α =0. Experimental signature The interference pattern measured by the detector D A is I A ( ϕ )=Tr( ρ A |0〉〈0|), with ρ A =Tr BC | ψ 〉〈 ψ | the reduced density matrix of photon A. The data can be postselected according to the outcome c resulting in I A| c . The intensity (signal) measured by detector D A for c =0 (and no post-selection on b ) is: giving the visibility A similar calculation gives the visibility for c =1 The full intensity measured by detector D A (without postselecting on c ) is and the corresponding visibility Thus the visibility of detector D A gives information about the entanglement of the BC pair. We now calculate the visibilities predicted by a non-trivial HV theory that is assumed to satisfy the three classical assumptions. Using equation (26), we rewrite the counting statistics as For the product probability distribution above, we get for j =0, 1 separately, where . As a result, giving for the visibilities in HV theories. How to cite this article: Ionicioiu, R. et al. Is wave–particle objectivity compatible with determinism and locality? Nat. Commun. 5:4997 doi: 10.1038/ncomms5997 (2014).